A universal description of ultraslow glass dynamics The dynamics of glass is of importance in materials science but its nature has not yet been fully understood. Here we report that a verification of the temperature dependencies of the primary relaxation time or viscosity in the ultraslowing/ultraviscous domain of glass-forming systems can be carried out via the analysis of the inverse of the Dyre–Olsen temperature index. The subsequent analysis of experimental data indicates the possibility of the self-consistent description of glass-forming low-molecular-weight liquids, polymers, liquid crystals, orientationally disordered crystals and Ising spin-glass-like systems, as well as the prevalence of equations associated with the ‘finite temperature divergence’. All these lead to a new formula for the configurational entropy in glass-forming systems. Furthermore, a link to the dominated local symmetry for a given glass former is identified here. Results obtained show a new relationship between the glass transition and critical phenomena. The glass transition constitutes one of the outstanding problems of condensed matter physics [1] , with fundamental importance for many areas ranging from geophysics to modern food science and material engineering [2] , [3] , [4] , [5] . Over the last decades, an important progress in this field has been achieved, primarily because of the progress in the state-of-the-art experimental, theoretical and numerical insights. Hence, a conceptual breakthrough seems to emerge [6] , [7] , [8] , [9] , [10] , [11] , [12] , [13] , [14] , [15] , [16] , [17] , [18] . Recently, however, serious doubts regarding the most fundamental experimental artifact, namely the parameterization of viscosity η ( T ) or primary relaxation time τ ( T ) on approaching the glass temperature ( T g ), appeared [15] , [19] , [20] , [21] . The importance of this issue is related to the fact that it is often associated with a hypothetical link between the glass transition and critical phenomena physics, that is, the thrilling possibility of a new great unification within condensed matter physics [14] , [18] . Moreover, relations portraying the evolution of η ( T ) or τ ( T ) are often considered as a checkpoint for theoretical models [3] , [13] . Decades of studies have led to the prevailing conviction that the ultimate parameterization is possible via the Vogel–Fulcher–Tammann (VFT) equation [3] , [13] , [22] , [23] , [24] : where D T denotes the fragility strength coefficient and T 0 is the VFT singular temperature ( and ). However, by following the compelling analysis of 43 sets of τ ( T ) data for low-molecular-weight ultraviscous liquids, Hecksher et al. [15] recently concluded: ‘There is no compelling evidence for the VFT prediction that the relaxation time diverges at a finite temperature […] with a dynamic divergence of the VFT form lack a direct experimental basis…. we suggest that in the search for the correct theory for ultraviscous liquid dynamics, theories not predicting a dynamic divergence of the VFT form should be focused on’. McKenna [25] extended this outlook to the case of polymer glass formers. These findings were strengthened by the derivation by Mauro et al. [19] of the equation introduced empirically by Waterton [26] : The subsequent analysis of experimental data confirmed the advantage of the Waterton-Mauro (WM, called also MYEGA) equation without a ‘finite temperature divergence’ over the VFT one [11] , [19] , [20] , [21] , [27] . Thus, the question regarding τ ( T ) or η ( T ) portrayal seemed to be clarified. However, the problem becomes more complex if glass-forming liquid crystals (LCs) and orientationally disordered crystals (ODICs; plastic crystals) are also considered. For these materials, the prevalence of the ‘critical-like’ equation with the clear ‘finite temperature divergence’ was clearly shown [28] , [29] : where and : most often T g − T 0 ≈30–40 K and T g − T C ≈10–15 K . Surprisingly, the latter description seems to be applicable also for selected low-molecular-weight liquids and polymers [28] , [29] . Worth mentioning is that such dynamics is also commonly accepted for spin-glass-like (SGL) systems [5] , [28] . Remarkable is furthermore the approximate coincidence of power exponents in the mentioned systems, namely φ ≈9 for LC [28] , [29] , φ =9–15 in ODIC [28] , [29] and φ =9–12 in SGL [3] , [13] , [28] . In this respect, it is important to point out the link between anomalous dynamics in supercooled glass-forming systems and the cooperatively rearranged regions, introduced by the Adam and Gibbs (AG) model [3] , [13] , [30] , leading to the following output relation [30] : where Δ μ defines that the free-energy barrier between cooperatively rearranged region and S C is the configurational entropy related to the difference between the entropy of the metastable disordered supercooled system and the stable crystal state. Angell et al. [31] , [32] , [33] noted that the AG equation can be converted into the VFT one by assuming: for T 0 = T K , where the latter denotes the Kauzmann temperature [34] . Although equation (5) became popular in the semi-phenomenological analysis of supercooled glass formers [3] , [13] , some puzzling issues remain. Mauro [11] , [19] has shown that the ‘divergence-less’ equation (2) can also be derived from the AG dependence by omitting equation (5) for the configurational entropy. Moreover, the analysis of experimental data indicated that the coincidence between T 0 and T K may be limited [35] . Eckmann and Procaccia [36] showed that for a soft potential based model, the configurational entropy can stay positive for , concluding that the Kauzmann temperature may not exist. Particularly noteworthy is that the parameterization of τ ( T ) or η ( T ) via ‘finite temperature divergence’ relations was used as an important argument to support the hypothesis, which correlates the glass transition with a hidden phase transition below T g . For instance, Colby [16] suggested that equation (3), with exponent φ =9, may be ‘universal’ for glass-forming low–molecular-weight liquids and polymers, although for some of them, a multiplicative factor exp( E/kT ) should be included. The ‘critical-like’ divergence was associated with a hypothetical phase transition at T C < T g , linked to the correlation length ξ ( T )= ξ 0 ( T − T C ) − v with (refs 16 , 17 ). However, a subsequent thorough analysis of τ ( T ) experimental data did not confirm the suggested superior-fitting features [28] , [29] , [37] . Notwithstanding, there are several low-molecular-weight and polymeric glass formers for which the behaviour suggested by Colby holds surprisingly well [28] , [29] . It is worth mentioning that in 2010, Tanaka et al. [18] carried out an in-depth simulation analysis of six glass-forming systems and stated: ‘Our results suggest a far more direct link than thought before between glass transition and critical phenomena. Indeed, the glass transition may be a new type of critical phenomenon where a structural order parameter is directly linked to slowness’. Tanaka et al. [18] linked the ‘pretransitional’ behaviour of the relaxation time to the Ising-like critical power-law divergence of the correlation length towards the ideal glass transition with the exponent , where d defines the spatial dimensionality. This led to the VFT-type equation . Tanaka et al. [18] , further suggested that glass transition may be encountered in the ‘Ising universality class for systems with a non-conserved order parameter’. At this point, some basic concepts of critical phenomena physics are worth recalling [38] , [39] . The pretransitional behaviour for different physical magnitudes ( X ( T )) is described by the relation X ( T ) | T − T C | λ , where the values of critical exponents ( λ ) are universal and depend solely on the dimensionality of the order parameter, the space dimensionality and the range of interactions. The symmetry is playing an essential role, whose changes are quantified by the order parameter. Microscopically, different systems can be ascribed in universality classes. It is also worth to bear in mind that the physics of critical phenomena is considered one of the greatest ‘unification’ successes in condensed matter physics of the 20th century [2] , [38] , [39] . To the best of the authors’ knowledge, no clear manifestation of the above fundamental features for the glass-transition phenomenon has been reported so far. This paper aims to fill this gap and resolve the Gordian knot of the τ ( T ) or η ( T ) evolution on approaching the glass transition. Fragility and the Dyre–Olsen temperature index The Super-Arrhenius (SA) evolution of relaxation time or viscosity in the ultraslowing/ultraviscous domain can be generally expressed as , where stands for the normalized apparent activation energy (AAE) and R denotes the gas constant [3] , [13] . The departure from the simple Arrhenius behaviour with E a =const is characterized by the fragility coefficient ( m ), introduced by Angell et al. [40] , [41] as the metric at the normalized plots log 10 τ or log 10 η versus T g /T : Although the fragility coefficient m provides a metric for glass-forming liquids within a wide diversity of materials, it is not the only parameter of this type [3] , [13] . A decade ago, Dyre–Olsen (DO) [42] noted the formal importance of the Grüneisen parameter ( γ ) [43] : It indicates that if the restoring force acting on an atom is non-linear in displacement, the individual phonon frequency ω i changes with the volume of crystal V , and parameter γ reaches a transition from zero (linear displacement) to γ >0 (ref. 43 ). In the SA domain, the AAE increases with a decreasing temperature, allowing a dramatic increase from constant values to , hence giving rise to a non-linear behaviour in the log 10 τ versus 1/ T representation. This formal similarity allowed to propose the metric of the SA behaviour by the ‘Grüneisen-style’ activation energy temperature index [42] : The DO temperature index can serve as the alternative metric of fragility, which can be also presented as , where and denote the apparent activation enthalpy [44] . Assuming the hypothetical ‘universal’ value for the prefactor τ 0 =10 −14 s (refs 3 , 13 , 15 ), one obtains: , for τ ( T g )=10 2 s and τ 0 =10 −14 s. Subsequently, taking into account the recent suggestion that 16< m <175 (ref. 45 ), one can estimate: . It is noteworthy that in 1997, Simon et al. [46] indicated the upper fragility limit m =214, yielding I DO ( T g )=12.375. Very recently, McKenna [47] indicated that if T 0 is an ideal glass transition, the value of m evaluated at T = T 0 = T g would tend towards infinity for all materials. The same can be expected for I DO ( T g ). Heksher et al. [15] showed that the analysis of I DO ( T ) may represent a decisive tool for testing the validity of the given equation for fitting τ ( T ) experimental data in low-molecular-weight glass-forming ultraviscous liquids. To quantify how exactly the VFT and the popular Bässler–Avramov [48] , [49] (BA) equations describe the data, they compared experimental and ‘theoretical’ values of I DO ( T ), namely [15] : Derivations of I DO ( T ) for equations (2) and (3) are presented in the Methods section. In the ultraslowing domain, near T g , they are as follows: A glimpse on equations (9) and (10) shows that reciprocals of DO indexes yield a linear dependence , namely: The discussed evolutions of DO indexes are shown graphically in Fig. 1 . Two characteristic features are worth mentioning, namely: and . It is worth stressing that while the physics associated with the fragility index m has been very broadly discussed [3] , [13] , [15] , [20] , [31] , [40] , [41] , [42] , [43] , [44] , [45] , [50] , [51] , the meaning and properties of the DO index is poorly explored so far [15] , [42] . 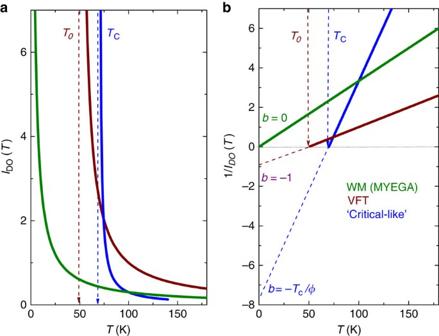Figure 1: Evolution of the DO temperature index for different equations portrayingτ(T) behaviour. (a,b) Evolutions of DO index for the WM (MYEGA) (green line), VFT (wine line) and ‘critical-like’ dependences (blue line). The omitted BA equation yields a horizontal line. Figure 1: Evolution of the DO temperature index for different equations portraying τ ( T ) behaviour. ( a , b ) Evolutions of DO index for the WM (MYEGA) (green line), VFT (wine line) and ‘critical-like’ dependences (blue line). The omitted BA equation yields a horizontal line. Full size image For the estimation of I DO ( T ), the evolution of E a ( T ) has to be determined. This, however, constitutes a notable issue. Hecksher et al. [15] calculated E a ( T ) from the SA relation, assuming τ 0 =10 −14 s as an ‘universal averaged’ value of the prefactor. However, in the systems analysed in this paper τ 0 =10 −11 s÷10 −16 s (refs 28 , 29 , 44 ). In the Methods section, we present a novel way of determining E a ( T ), avoiding the biasing influence of poorly estimated values of the prefactor τ 0 for the given system. Experimental data analysis This paper focuses on the ultraslow/ultraviscous domain as in Hecksher et al. [15] , for or , which usually occurs for (refs 50 , 51 , 52 , 53 ). By heating above T B , the so-called dynamic cross-over occurs. The discussion on recent advances regarding this phenomenon can be found in Martinez-Garcia et al. [52] The analysis of experimental data presented below does not only cover the most often discussed supercooled low-molecular-weight liquids (L) and multimeric and polymeric (P) glass formers as in Hecksher et al. [15] , but also LCs, plastic crystals (ODICs) and SGL systems. The analysis is based on 16 selected sets of τ ( T ) experimental data representing these types of glass-forming systems. However, to clarify the discussion, the key results are presented for a smaller number of characteristic systems. They are L including diethyl phthalate (DEP), glycerol, sorbitol, ethanol [28] , [54] , P including EPON 828 and polystyrene ( M W =700) (refs 28 , 55 ), ODIC ( plastic crystal ) including C7-OH, C8-OH (ref. 53 ), CNc6 (ref. 57 ), CNadm [58] , [59] and NPaNPG 0.3 (ref. 56 ), and SGL including ferrofluid liquid, with 5% solution of single-domain particles of the amorphous alloy Fe 1− x C x ( x =0.2–0.3) (ref. 57 ). Details regarding all tested systems are collected in the Supplementary Table S1 . The presented analysis is focused on the primary relaxation time τ ( T ), because the modern broad-band dielectric spectroscopy can yield sets of high precision and consistent experimental data [3] , [13] . For the presentation of experimental data, we apply the linearized derivative-based analysis introduced in Drozd-Rzoska and Rzoska [44] . The VFT equation allows the following transformation of τ ( T ) data: For the critical-like equation (3): where stands for the normalized apparent enthalpy. The linear behaviour of equations (12) and (13) show the valid temperature domain of the VFT and ‘critical-like’ equations. The subsequent linear regression fit can yield optimal values of relevant parameters [44] . Results of such analysis for selected systems are shown in Fig. 2a–e . It is visible that a clear ‘critical-like’ parameterization is preferred for all LC rod-like compounds, as well as for sorbitol, ethanol and polystyrene ( Fig. 2b ). This behaviour can be linked to the uniaxial structure of molecules, which may lead to the local orientational symmetry (OS) arrangements [28] . The ‘critical-like’ behaviour also dominates the dynamics of plastic crystals (ODICs) [28] , [29] , where a positional symmetry (PS) is a fundamental feature ( Fig. 2a ). Regarding EPON 828, glycerol and DEP, the critical-like parameterization definitively fails ( Fig. 2c ). Because these compounds cannot be linked neither to OS nor to PS cases, we assigned them as no-symmetry (NS) compounds. 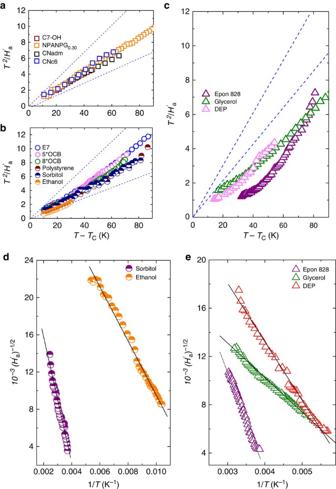Figure 2: Linearized derivative-based presentation ofτ(T) data. Results of the linearized, derivative-based transformations44ofτ(T) experimental data, withand. (a–c) Refer to (equations (3) and (13)). (d,e) Refer to the VFT dependence (equations (1) and (12)). The domains of the validity of the given description are shown via the linear behaviour. The blue dashed lines in a–c stand for ‘terminal critical exponents’φ=8 and 12, respectively. Figure 2: Linearized derivative-based presentation of τ ( T ) data. Results of the linearized, derivative-based transformations [44] of τ ( T ) experimental data, with and . ( a – c ) Refer to (equations (3) and (13)). ( d , e ) Refer to the VFT dependence (equations (1) and (12)). The domains of the validity of the given description are shown via the linear behaviour. The blue dashed lines in a–c stand for ‘terminal critical exponents’ φ =8 and 12, respectively. Full size image For ‘NS’ glass formers, the VFT equation fits the experimental data fairly well as shown in Fig. 2e . It is noteworthy that for ethanol and sorbitol, both equations (1) and (3) seem to offer the acceptable parameterization ( Fig. 2b ). For a further insight into the optimal τ ( T ) parameterization, an analysis exploring behaviour has been carried out ( Fig. 3 and equation (11)). It is visible that for none of the tested compounds, the evolution expected for BA [49] ( ) or WM [19] ( ) relations take place. Solely, patterns expected for the VFT or the ‘critical-like’ description occurs. Experimental results show that such patterns are associated with three ‘terminal, convergence’ cases: (i) , for ODICs and SGL (PS case); (ii) n ≈1.53, for all LCs and also low-molecular-weight sorbitol, propanol and polystyrene (OS case); (iii) n ≈1, for DEP, EPON 828 and glycerol (NS case). Worth to mention is that the points (i) and (ii) are related to approximately the same value of the ‘critical’ exponent φ =8.5~12 in equation (3), being remarkable that the plot allows to separate OS and PS cases. 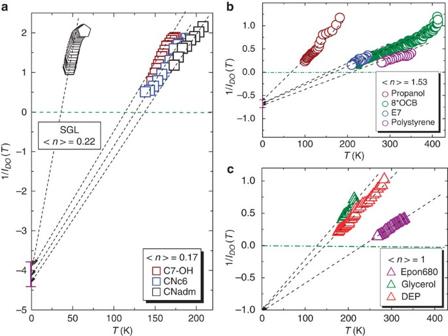Figure 3: Reciprocals of the experimental DO temperature index. The temperature evolution of the inverse DO index for tested glass-forming materials given in the figure. The analysis disentangles three representative cases: (a) the ‘PS’ (ODICs and SGL); (b) the ‘OS’ (LC, propanol and polystyrene); and (c) the lack of dominant symmetry (NS). Note the convergence emerging for 1/IDO(T=0). Figure 3: Reciprocals of the experimental DO temperature index. The temperature evolution of the inverse DO index for tested glass-forming materials given in the figure. The analysis disentangles three representative cases: ( a ) the ‘PS’ (ODICs and SGL); ( b ) the ‘OS’ (LC, propanol and polystyrene); and ( c ) the lack of dominant symmetry (NS). Note the convergence emerging for 1/ I DO ( T =0). Full size image A summary of the analysis covering 16 glass-forming systems is presented in Fig. 4 and in the Supplementary Table S1 . Apart from the already-mentioned manifestation of three ‘characteristic’ values of the coefficient n , which can be related to the local symmetry, two more issues are notable. First, the clear access of the SGL system to the PS group, together with ODICs. Second, the ‘intermediate’ cases between three characteristic values of the coefficient n . For ethanol, the coefficient is n ≈1.2, whereas for propanol, being a ‘longer’ and thus more uniaxial compound and from the same homologous series, the coefficient is n ≈1.5, as for LCs and polystyrene. One of the ‘intermediate’ cases is cyclooctanol (plastic crystal), for which n ≈0.8. In this case, the discrepancy may be linked to some distortion from the optimal positional ordering. 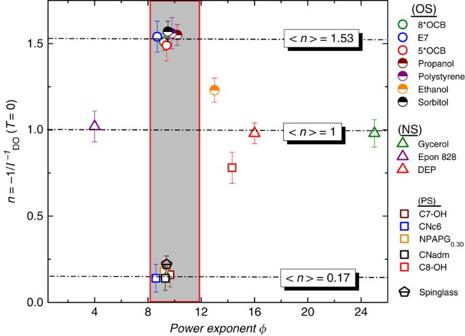Figure 4: Coefficientnversus the exponentφ. Experimental dependencies of the symmetry coefficient (n) versus the power exponentφ(equations (3) and (13)). For systems with the dominant VFT parameterization the exponent has been estimated as the terminal caseφ(T→Tg). Convergence values of the coefficient (n) related to VFT or ‘critical-like’ behaviours are indicated. The separation of OS and PS cases indicates the role of the symmetry. Figure 4: Coefficient n versus the exponent φ . Experimental dependencies of the symmetry coefficient ( n ) versus the power exponent φ (equations (3) and (13)). For systems with the dominant VFT parameterization the exponent has been estimated as the terminal case φ ( T → T g ). Convergence values of the coefficient ( n ) related to VFT or ‘critical-like’ behaviours are indicated. The separation of OS and PS cases indicates the role of the symmetry. Full size image Consequences for the configurational entropy Assuming the validity of equation (4), recalling equation (18) from Martinez-Garcia et al. [52] and the definition of the DO index by equation (8), the following relation can be formulated: By applying experimental findings from the previous section, the above equation can be written as: The latter directly yields the following solution: where the ‘singular’ temperature can be defined as and the power exponent as . Equation (16) represents a new generalized dependence for the evolution of the configurational entropy of glass-forming liquids, allowing to construct the normalized/scaling plot shown in Fig. 5 . 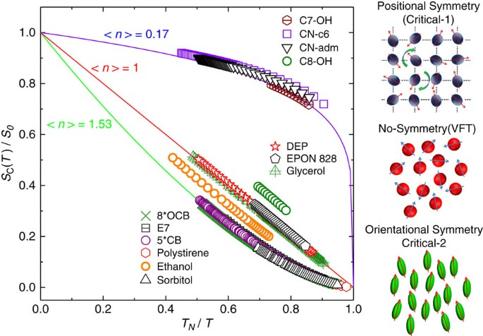Figure 5: Scaling configurational entropy plot. It shows the experimental evolution of the normalized structural entropy for selected experimental ultraslowing systems. The analytic evolution related to PS, NS and OS patterns (solid curves) is coupled to different ‘universal’ values of the coefficient exponentn=−1/IDO−1(T=0). The related symmetries are also illustrated. Figure 5: Scaling configurational entropy plot. It shows the experimental evolution of the normalized structural entropy for selected experimental ultraslowing systems. The analytic evolution related to PS, NS and OS patterns (solid curves) is coupled to different ‘universal’ values of the coefficient exponent n =−1/ I DO −1 ( T =0). The related symmetries are also illustrated. Full size image The scaling Fig. 5 covers the variety of ultraslowing glass-forming systems ranging from low-molecular liquids and polymers to plastic crystals, LCs and SGLs. Clearly visible are three characteristic (universal?) values of the power exponent: n ≈1.53, n =1 and n ≈0.17, which can be linked to different dominating molecular symmetries, as shown in the right part of Fig. 5 . Worth to mention is also that equation (16) has been derived by the solution of the first-order differential equation (15), without underlying assumptions that were used in the derivation of equation (5). The latter is recovered for n =1. It is also noteworthy that equation (16) indicates a possible link between the ‘critical’ temperature ( T C ) in equation (3) and the VFT singular temperature ( T 0 ) in equation (1)). In the year 2008, Hecksher et al. [15] boosted the discussion regarding one of the most fundamental experimental artifacts within glass-transition physics, namely the validity of the VFT equation, the existence of the ‘final temperature divergence’ < T g , and the ultimate way of τ ( T ) or η ( T ) parameterization. This discussion and subsequent papers [28] , [29] , [52] have indicated that parameterizations not associated with a ‘finite temperature divergence’ may be crucial. All these findings indirectly questioned the connection between the glass transition and a hidden phase transition below T g . However, parallel studies exploring the linearized derivative and distortion sensitive analysis led to a clear proof that the ‘critical-like’ description with a finite temperature divergence may be optimal for liquid crystalline glass formers, plastic crystals (not tested in Erwin and Colby [17] ) and even for selected low-molecular liquids and polymers [27] , [28] . This paper shows that the ‘finite temperature divergence’ in ultraslowing glass-forming systems on approaching T g may be feasible not only for low-molecular-weight liquids and polymers but also for LCs, plastic crystals and even SGL systems. Surprisingly, a consistency seems to be possible, despite the fact that a single equation for portraying the dynamics in the ultraslowing domain for an arbitrary glass former may not exist. It is worth stressing that the optimal parameterization via the VFT equation should be considered solely for selected compounds, and other systems such as parameterization is inherently non-optimal. This fact ought to be taken into account when validating different equations for portraying the τ ( T ) or η ( T ) experimental behaviour. We would like to stress the results of the analysis focused on BA [48] , [49] and WM (MYEGA) equations [11] , [19] , [26] without the finite temperature divergence. Worth to mention is also a group of further equations of such type [2] , [3] , [13] , [15] , which should be tested in the future. In conclusion, the obtained key forms for τ ( T ) or η ( T ) parameterization can be linked to predefined values of the parameter/exponent , as well as to the dominating local symmetry. They are clearly associated with a finite temperature divergence below the glass temperature. All these results indicate qualitatively new links between glass transition and critical phenomena. Analysis of experimental data The analysis of ‘dynamic’ experimental data employing higher-order derivatives of τ ( T ) or η ( T ) experimental data is most often avoided due to scatter associated with the inherent experimental error. In this paper, this basic issue has been overcome due to the novel implementation of Savitzky–Golay (SG) filtering procedure introduced in Martinez-Garcia et al. [52] Determination of the AAE from τ ( T ) experimental data For estimating the DO temperature index ( I DO ( T )), the experimental evolution of the AAE is needed (equation (8)). So far, it was calculated from the ‘general’ apparent SA equation via , assuming for τ 0 =10 −14 s, which is most often considered as the ‘typical’ or ‘universal’ value, at least for ultraviscous liquids. Notwithstanding, there is clear evidence that the value of τ 0 ranges from 10 −11 –10 −16 s (ref. 49 ). The erroneous value τ 0 for a given experimental system can notably influence estimations of E a ( T ). In this paper, experimental values of E a ( T ) were calculated in a novel way, avoiding τ 0 -related problems. The AAE was calculated via . Ultimate estimation was supported by the SG filtering procedure. Subsequently, the following ‘general’ first-order differential equation was solved: The ‘noise-related’ scatter of the calculated E a ( T ) values was minimized by the SG filtering procedure for each tested glass-forming system. In a next step, the DO was calculated via the equation (8). Derivations of the DO temperature indexes for selected equations describing τ ( T ) or η ( T ) evolutions The form of I DO ( T ) for VFT equation (1) and BA relation can be found in Erwin and Colby [17] . The DO temperature index for the WM (MYEGA) equation can be obtained by linking equation (2), the SA equation and I DO ( T ) definition (equation (8)): Forms of I DO ( T ) for the critical-like case in the ultraslowing/ultraviscous dynamic domain can be obtained by linking equation (3) and the general SA dependence : This work focuses on the ultraviscous/ultraslowing dynamic domain close to T g , that is, for T → T C , hence: The latter equation can be re-written as: The function can be expanded into the Taylor series because of its inherent features ( ) if | δ ( T )−1|≤1. This condition is valid for ultraslowing ODICs, LCs and SGL systems tested in this paper. Taking this into account, one obtains: Then, recalling I DO ( T ) definition (equation (8)): The evolutions of and are presented graphically in Fig. 6 . 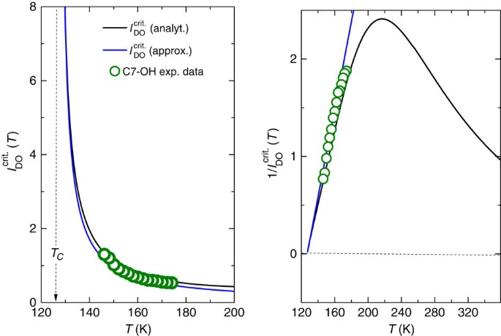Figure 6: Analytic and approximated evolution of the ‘critical-like’ DO temperature index. Evolutions ofIDOcrit.(analyt.) (black curve),IDOcrit.(approx.) (blue curve) and their reciprocals (right side), compared with the empirical DO index for C7-OH (ODIC, plastic crystal) where the critical-likeτ(T) evolution is optimal. Figure 6: Analytic and approximated evolution of the ‘critical-like’ DO temperature index. Evolutions of I DO crit. (analyt.) (black curve), I DO crit. (approx.) (blue curve) and their reciprocals (right side), compared with the empirical DO index for C7-OH (ODIC, plastic crystal) where the critical-like τ ( T ) evolution is optimal. Full size image The analytic form of the index is given in the bracket in equation (24) and shown graphically in Figure 6 , together with the approximation . This figure is supplemented by the experimental DO index for C7-OH (ODIC; plastic crystal) where the critical-like parameterization of τ ( T ) is optimal (see Fig. 2 ). The validity of for portraying experimental data in the ultraslowing domain (below T B ) is clearly visible. How to cite this article: Martinez-Garcia, J. C. et al. A universal description of ultraslow glass dynamics. Nat. Commun. 4:1823 doi: 10.1038/ncomms2797 (2013).